Mutations in Alström protein impair terminal differentiation of cardiomyocytes Cardiomyocyte cell division and replication in mammals proceed through embryonic development and abruptly decline soon after birth. The process governing cardiomyocyte cell cycle arrest is poorly understood. Here we carry out whole-exome sequencing in an infant with evidence of persistent postnatal cardiomyocyte replication to determine the genetic risk factors. We identify compound heterozygous ALMS1 mutations in the proband, and confirm their presence in her affected sibling, one copy inherited from each heterozygous parent. Next, we recognize homozygous or compound heterozygous truncating mutations in ALMS1 in four other children with high levels of postnatal cardiomyocyte proliferation. Alms1 mRNA knockdown increases multiple markers of proliferation in cardiomyocytes, the percentage of cardiomyocytes in G2/M phases, and the number of cardiomyocytes by 10% in cultured cells. Homozygous Alms1 -mutant mice have increased cardiomyocyte proliferation at 2 weeks postnatal compared with wild-type littermates. We conclude that deficiency of Alström protein impairs postnatal cardiomyocyte cell cycle arrest. Mammalian cardiac development requires continuous proliferation of cardiomyocytes throughout gestation [1] , [2] . During the perinatal period, cardiomyocyte proliferation rapidly declines, and the majority of cardiomyocytes undergo cell cycle arrest with terminal differentiation [3] , [4] . Postnatal arrest of the cardiomyocyte cell cycle is a key event for maturation of the mammalian heart, but this process is poorly understood [3] . A recent report highlights the role of the homeodomain transcription factor, Meis1, as a critical regulator of postnatal cardiomyocyte cell cycle arrest, though this process remains incompletely understood [5] . Unusual human phenotypes sometimes offer the opportunity to understand normal development or disease pathogenesis, if the cause can be determined. Mitogenic cardiomyopathy is a rare form of paediatric cardiomyopathy characterized by persistent markers of mitotic activity in cardiomyocytes [6] . Among five previously reported infants with this condition, there were two pairs of siblings, one of whom had parental consanguinity supporting a recessive genetic disorder. Although transgenic models of postnatal cardiomyocyte replication have been developed, no naturally inherited conditions have previously been characterized in humans that are associated with delayed postnatal cardiomyocyte cell cycle arrest [7] , [8] . Recognition and characterization of such a disorder has the potential to identify important regulators of the transition of cardiomyocytes from active proliferation to terminal differentiation. Here we identify ALMS1 mutations in two siblings and four previously reported infants with ‘mitogenic cardiomyopathy.’ We show that small interfering RNA-induced (siRNA-induced) knockdown of murine Alms1 increases cell cycle progression in cultured neonatal murine cardiomyocytes, and Alms1 knockdown also increases the number of induced cardiomyocytes in counting experiments. Mice with targeted mutation of Alms1 have delayed exit from active cell cycle progression, further supporting an important role for ALMS1 in regulating postnatal cardiomyocyte cell cycle arrest. Evaluation of the proband and her sibling We identified two infant siblings with neonatal heart failure, both of whom required cardiac transplantation. The proband was normal at birth, and she had no other manifestations of Alström syndrome before transplantation, which was performed at 3 months of age. The proband’s only sibling underwent cardiac transplantation at age 5 months for similar cardiac dysfunction. Intracranial bleeding complicated her post-operative course, and she died 1 month later. Cardiac evaluations of both parents were normal. We visualized mitotic cardiomyocytes with antibodies against phosphorylated histone H3 (PH3, a marker for M-phase [9] ) and cardiac troponin T (cTnT) ( Fig. 1a,b,d ), and as well as wheat germ agglutinin (WGA) to distinguish cell boundaries ( Fig. 2 ). Using an unbiased double-blinded approach for quantification of proliferating myocytes, we quantified PH3-positive cardiomyocytes in multiple fields from the proband and three age-matched controls with heart failure. The amount of PH3-positive cardiomyocytes was higher in the proband than in the controls (114.3±31.3 mm −2 ( N =4) versus 0.28±0.07 mm −2 ( N =12), Student’s t -test, mean±s.e.m., respectively). To validate the high number of proliferating cardiomyocytes in the proband, we stained with antibodies against phospho-aurora kinases (PAKs) A, B and C. PAK A/B/C are important regulators of karyokinesis and cytokinesis, and localization of PAK-B to the cleavage furrow is required for establishing cytokinesis [10] . Aurora kinases are essential for formation of the mitotic spindle, separation of centrosomes and assembly of the cleavage furrow during pro-, meta-, ana- and telophase of mitosis [10] , [11] , [12] . Immunostaining for PAK confirmed an increase in the number of positively stained cardiomyocytes in multiple fields from the proband compared with the age-matched controls with heart failure (12.2±2.6 mm −2 ( N =4) versus ≤0.02±0.01 mm −2 ( N =12), Student’s t -test, mean±s.e.m., respectively) ( Fig. 1e,f ). 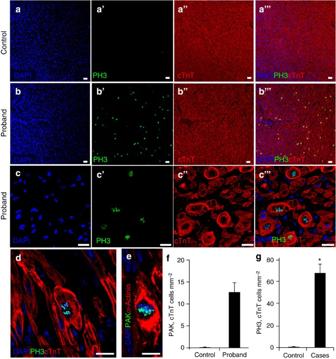Figure 1: Increased cardiomyocyte proliferation in people withALMS1mutations. (a,b) Representative confocal images of the proband heart versus age-matched control; PH3 (green), troponin T (red) and DAPI (blue). (c) Higher magnification confocal images of PH3-positive cardiomyocytes in the proband; PH3 (green), troponin T (red) and DAPI (blue). (d) Additional high-magnification confocal image of a PH3-positive cardiomyocyte in the proband; PH3 (green), troponin T (red) and DAPI (blue). (e) Phospho-aurora kinase (PAK) staining (green) is present in a dividing cardiomyocyte nucleus in the proband; PAK (green), α-sarcomeric actinin (red) and DAPI (blue). (f) The number of PAK-positive cardiomyocytes in the heart of the proband was compared with three age-matched controls with failing ventricles. (g) The number of PH3-positive cardiomyocytes in affected individuals was compared with three age-matched controls with failing ventricles. Error bars represent s.e.m. Scale bars, 10 μm. ‘*’ refers toP<0.01 using unpaired Student'st-test. (a,b,c) DAPI; (a',b',c') PH3; (a'',b'',c'') cTnT; (a''',b''',c''') merged images with DAPI, PH3, and cTnT. Figure 1: Increased cardiomyocyte proliferation in people with ALMS1 mutations. ( a , b ) Representative confocal images of the proband heart versus age-matched control; PH3 (green), troponin T (red) and DAPI (blue). ( c ) Higher magnification confocal images of PH3-positive cardiomyocytes in the proband; PH3 (green), troponin T (red) and DAPI (blue). ( d ) Additional high-magnification confocal image of a PH3-positive cardiomyocyte in the proband; PH3 (green), troponin T (red) and DAPI (blue). ( e ) Phospho-aurora kinase (PAK) staining (green) is present in a dividing cardiomyocyte nucleus in the proband; PAK (green), α-sarcomeric actinin (red) and DAPI (blue). ( f ) The number of PAK-positive cardiomyocytes in the heart of the proband was compared with three age-matched controls with failing ventricles. ( g ) The number of PH3-positive cardiomyocytes in affected individuals was compared with three age-matched controls with failing ventricles. Error bars represent s.e.m. Scale bars, 10 μm. ‘*’ refers to P <0.01 using unpaired Student's t -test. ( a , b , c ) DAPI; ( a' , b' , c' ) PH3; ( a'' , b'' , c'' ) cTnT; ( a''' , b''' , c''' ) merged images with DAPI, PH3, and cTnT. 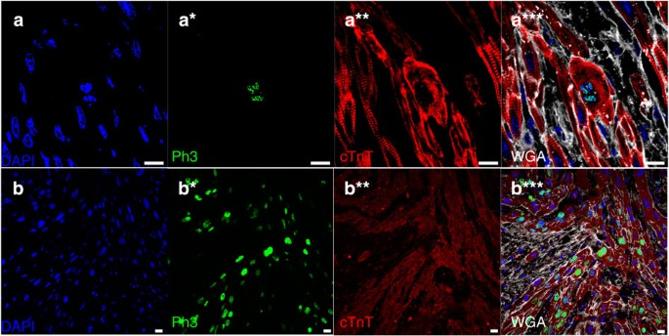Figure 2: PH3-positive cardiomyocytes in the proband and another affected individual. Additional representative confocal microscopic images from the heart of the proband (a) and another individual with mitogenic cardiomyopathy (b) have high levels of phosphohistone-H3 (PH3) positivity. Images were obtained with confocal microscopy using immunostaining for Ph3 (green), α-sarcomeric actinin or troponin T (red), WGA (white) to outline cell boundaries and DAPI (blue) to highlight nuclei. (a,b) DAPI; (a*,b*) Ph3; (a**,b**) cTnT; (a***,b***) merged images with DAPI, Ph3, cTnT and WGA. Scale bars, 10 μM. Full size image Figure 2: PH3-positive cardiomyocytes in the proband and another affected individual. Additional representative confocal microscopic images from the heart of the proband ( a ) and another individual with mitogenic cardiomyopathy ( b ) have high levels of phosphohistone-H3 (PH3) positivity. Images were obtained with confocal microscopy using immunostaining for Ph3 (green), α-sarcomeric actinin or troponin T (red), WGA (white) to outline cell boundaries and DAPI (blue) to highlight nuclei. ( a , b ) DAPI; ( a *, b *) Ph3; ( a **, b **) cTnT; ( a ***, b ***) merged images with DAPI, Ph3, cTnT and WGA. Scale bars, 10 μM. Full size image The proband underwent clinical genetic testing to determine the cause of her cardiomyopathy with a resequencing array [13] . Analysis of MYH7, MYBPC3, TNNT2, TNNI3, TPM1, ACTC, LMNA, SGCD, EMD, DES, LDB3, ACTN2, CSRP3, TCAP, VCL, TAZ, PLN, ABCC9, and CTF1 showed no apparent cause for cardiomyopathy. Next, we performed whole-exome sequencing using DNA obtained from the affected proband and both of her parents. With the presumption of a recessive disorder, we focused on missense, nonsense or splice site variants that were likely to be compound heterozygote mutations in the affected offspring, as the ethnicity of the parents was geographically distant (northern European and Southeast Asian). Variants present in dbSNP131 or the 1,000 genomes pilot April 2010 data set were filtered out. After this level of filtering, six genes with compound missense variants and one gene with compound heterozygote frameshift insertion/deletion remained ( Table 1 ). The 1,000 genomes November 2010 data were subsequently available, and three of these genes with previously novel compound heterozygous missense variants were filtered. Sanger sequencing confirmed novel DNA variants in each of the remaining four genes. The absence of one or both variants in the affected sibling led to filtering of two additional genes. FERMT1 had two novel missense alleles (p.Arg98Cys and p.Val519Leu) that were present in each of the affected individuals. These novel variants in FERMT1 were prioritized lower than ALMS1 because Arg98 is not highly conserved (Cys in Danio rerio ), and because valine and leucine are both neutral nonpolar amino acids (Grantham score 32); both variants are present at low levels in the NHLBI Exome Variant Server. We identified and confirmed two heterozygous ALMS1 mutations in the proband and her sibling, both of which result in frameshift and premature termination (c.1794_1801dup8 in exon 8 and c.11116_11134del19 in exon 16). Mutations in ALMS1 are known to cause Alström syndrome, a recessive systemic disorder [14] . The c.11116_11134del19 mutation was previously reported in a patient with Alström syndrome [15] . Each parent harboured one of the mutant ALMS1 alleles. Alström syndrome (Online Mendelian Inheritance in Man no. 203800) is a recessive ciliopathy caused by ALMS1 mutations and characterized by childhood truncal obesity, insulin-resistant diabetes mellitus, sensorineural hearing loss, retinal degeneration and systemic fibrosis affecting multiple organs (kidney, liver, lung and heart) [16] , [17] . Cardiomyopathy manifests in approximately two-thirds of affected individuals, and it can precede all other manifestations, obscuring the diagnosis of Alström [18] , [19] . We hypothesized that the mutations in ALMS1 caused the delayed terminal differentiation of cardiomyocytes. Table 1 Filtered exome-sequencing results. Full size table ALMS1 mutations in similarly affected infants To extend these findings, we sequenced ALMS1 in four additional infants (two sibling pairs) with mitogenic cardiomyopathy, from whom DNA was available [6] . We identified homozygous or compound heterozygous mutations in each of them ( Table 2 ). For all cellular and immunohistochemical quantifications, unpaired two-tailed Student’s t -test, type II, was used for data analysis and P ≤0.5 was considered as significant. Using the same double-blinded quantification method described above, we quantified PH3-positive cardiomyocytes in three affected individuals (one from each sibling pair) and compared with three age-matched controls with heart failure, and found it to be higher in the affected children (67.3±8.6 mm −2 compared with 0.28±0.07 mm −2 , respectively, N =3, mean±s.e.m., P <0.01; Fig. 1g ). Accordingly, DNA content in dividing cardiomyocytes was 1.9-fold greater in PH3-positive myocytes than in non-dividing cells, confirming that PH3-positive myocytes are undergoing mitosis ( Fig. 3 ). Table 2 Mutations in ALMS1 in people with mitogenic cardiomyopathy. 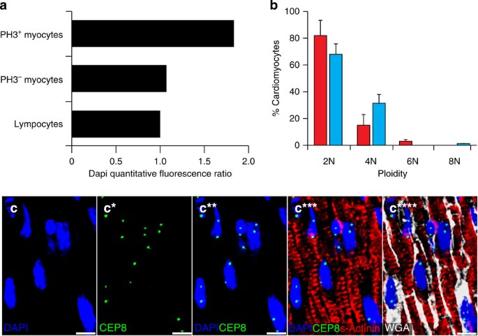Figure 3: Human cells analysed for ploidy status. (a) The DNA content in dividing cardiomyocyte nuclei was compared with non-dividing nuclei (both cardiomyocytes and non-cardiomyocytes) in the proband using quantitative confocal laser cytometry with DAPI nuclear staining. The ratio of DNA in nuclei from proliferating cardiomyocytes compared with non-proliferating (cardiomyocyte and lymphocyte) nuclei in the proband is 1.9, indicating predominantly 4N chromosomal content in these cells. (b) Summary of the ploidy analysis using centromeric probes for four affected individuals and two unaffected controls. Error bars indicate s.e.m. (c) An example of ploidy analysis using one of the centromere FISH probes for chromosome 8 (CEP8) in an affected individual. Colour staining is shown in the bottom left. Scale bars, 10 μM; these five panels are the same field with: (c) DAPI; (c*) CEP8; (c**) DAPI and CEP8; (c***) DAPI, CEP8 and sarcomeric actinin; and (c****) DAPI, CEP8, sarcomeric actinin and WGA. Full size table Figure 3: Human cells analysed for ploidy status. ( a ) The DNA content in dividing cardiomyocyte nuclei was compared with non-dividing nuclei (both cardiomyocytes and non-cardiomyocytes) in the proband using quantitative confocal laser cytometry with DAPI nuclear staining. The ratio of DNA in nuclei from proliferating cardiomyocytes compared with non-proliferating (cardiomyocyte and lymphocyte) nuclei in the proband is 1.9, indicating predominantly 4N chromosomal content in these cells. ( b ) Summary of the ploidy analysis using centromeric probes for four affected individuals and two unaffected controls. Error bars indicate s.e.m. ( c ) An example of ploidy analysis using one of the centromere FISH probes for chromosome 8 (CEP8) in an affected individual. Colour staining is shown in the bottom left. Scale bars, 10 μM; these five panels are the same field with: ( c ) DAPI; ( c *) CEP8; ( c **) DAPI and CEP8; ( c ***) DAPI, CEP8 and sarcomeric actinin; and ( c ****) DAPI, CEP8, sarcomeric actinin and WGA. Full size image Cardiomyocytes can undergo DNA replication without completing the cell cycle. Polyploidization occurs during early postnatal development and in response to myocardial stress [4] , [20] , [21] . We considered the possibility that ALMS1 deficiency could result in increased polyploidy. We applied centromeric fluorescence in situ hybridization (FISH) probes to determine the ploidy status in these infants with mitogenic cardiomyopathy. The percentage of 4N cardiomyocytes was 31.1±7.2% among affected individuals ( N =4) and 15.5±8.3% in the controls ( N =12), Student’s t -test, mean±s.e.m., P =0.26. Although we found cardiomyocytes that were polyploid (>4N), there was no difference between affected individuals (0.4%, N =4) and failing heart age-matched controls (0.6%, N =2) ( Fig. 3 ). Taken together, these results indicate that ALMS1 deficiency in cardiomyocytes does not lead to increased polyploidy. Alms1 knockdown increases cardiomyocyte cell cycling To confirm that ALMS1 loss is sufficient for extending the postnatal proliferative window of cardiomyocytes, we treated cultured neonatal mouse cardiomyocytes with Alms1 siRNA ( Supplementary Fig. 1 ). After 48 h, cells were stained with antibodies against Ki67 (a wide-ranging marker of proliferation) or Vybrant DyeCycle Ruby Stain (a marker of DNA content for determination of cell cycle; Invitrogen), together with cTnT, and analysed by flow cytometry. In ALMS1-deficient cardiomyocytes, Ki67-positive cardiomyocytes were 2.5-fold higher compared with control (4.2% versus 1.7%, respectively; N =8, Student’s t -test, P <0.05) ( Supplementary Fig. 2 ). Likewise, we observed more cells in G2/M phases after Alms1 knockdown compared with the control (13.3±1.8% versus 9.6±1.3%, mean±s.e.m., N =4, respectively, Student’s t -test, P <0.05) ( Fig. 4 ). We also analysed Ki67 expression in cells stained with the fibroblast marker Thy-1 (ref. 22 ) and found no significant difference between ALMS1-deficient cardiac fibroblasts compared with control (3.5±0.5% versus 2.9±0.8%, mean±s.e.m., N =4, respectively, Student’s t -test, P =0.55), indicating that the observed increase of cells in G2/M may be in cardiomyocytes. To determine whether the observed increase in G2/M was mediated by cardiomyocytes, we cultured neonatal mouse cardiomyocytes obtained from transgenic mice in which the α-myosin heavy chain (αMHC) promoter drives expression of green fluorescent protein (GFP), and thus only cardiomyocytes produce GFP [23] . After Alms1 knockdown, the number of GFP-positive cells in phases G2/M was increased compared with the control (11.3±1.0% versus 7.0±0.9%, mean±s.e.m., N =3, respectively, Student’s t -test, P <0.05) ( Fig. 5a ), indicating that ALMS1 deficiency leads to impaired cell cycle arrest in cardiomyocytes. 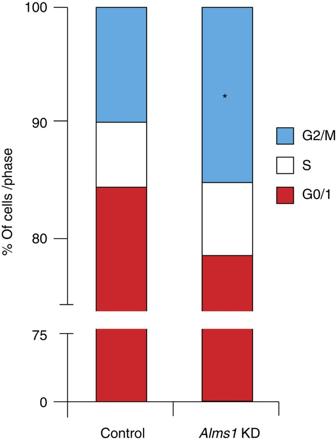Figure 4: Knockdown ofAlms1increases the number of cells in G2/M phases in cardiomyocyte-enriched cultures. Comparison of the percentage (%) of cells in different phases of cell cycle between control transfection andAlms1knockdown (KD) using siRNA; red=G0 or G1 phase; white=S phase; and blue=G2 or M phase. ‘*’ refers toP<0.05 using unpaired Student’st-test. Figure 4: Knockdown of Alms1 increases the number of cells in G2/M phases in cardiomyocyte-enriched cultures. Comparison of the percentage (%) of cells in different phases of cell cycle between control transfection and Alms1 knockdown (KD) using siRNA; red=G0 or G1 phase; white=S phase; and blue=G2 or M phase. ‘*’ refers to P <0.05 using unpaired Student’s t -test. 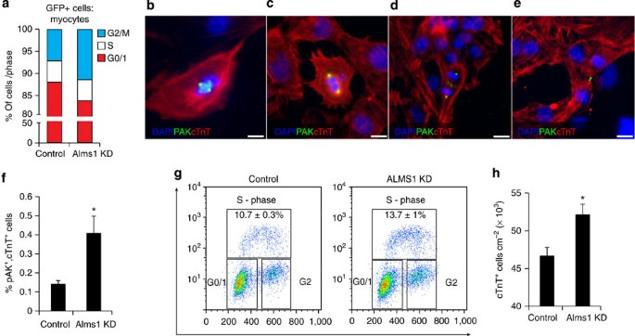Figure 5: Increased cardiomyocyte proliferation in cultured cells afterAlms1knockdown. (a) Comparison of αMHC-GFP-positive cardiomyocytes in different phases of cell cycle after control siRNA transfection compared withAlms1knockdown (KD) by siRNA; red=G0 or G1 phase, white=S phase, blue=G2 or M phase;N=3.Alms1KD increases the proportion of cells in G2/M phase (blue). (b–e) PAK-positive cardiomyocytes in different phases of mitosis; cTnT (red), PAK (green) and DAPI (blue);bis prophase,cis metaphase,dis anaphase, andeis telophase. (f) Flow cytometry of puromycin-selected cardiomyocytes (cTnT+cells) shows that afterAlms1KD, there is increased PAK expression compared with controls;N=3. (g) Scatter plot showing increased incorporation of EdU (yaxis) and increased DNA content by DAPI (xaxis) in puromycin-selected (cTnT+) cardiomyocytes withALMS1KD;N=15. (h) Total number of puromycin-selected cardiomyocytes afterAlms1KD is increased compared with controls;N=4. In all figures, ‘*’ refers toP<0.05 using Student’st-test. Error bars represent s.e.m. Scale bars, 5 μM. Full size image Figure 5: Increased cardiomyocyte proliferation in cultured cells after Alms1 knockdown. ( a ) Comparison of αMHC-GFP-positive cardiomyocytes in different phases of cell cycle after control siRNA transfection compared with Alms1 knockdown (KD) by siRNA; red=G0 or G1 phase, white=S phase, blue=G2 or M phase; N =3. Alms1 KD increases the proportion of cells in G2/M phase (blue). ( b – e ) PAK-positive cardiomyocytes in different phases of mitosis; cTnT (red), PAK (green) and DAPI (blue); b is prophase, c is metaphase, d is anaphase, and e is telophase. ( f ) Flow cytometry of puromycin-selected cardiomyocytes (cTnT + cells) shows that after Alms1 KD, there is increased PAK expression compared with controls; N =3. ( g ) Scatter plot showing increased incorporation of EdU ( y axis) and increased DNA content by DAPI ( x axis) in puromycin-selected (cTnT + ) cardiomyocytes with ALMS1 KD; N =15. ( h ) Total number of puromycin-selected cardiomyocytes after Alms1 KD is increased compared with controls; N =4. In all figures, ‘*’ refers to P <0.05 using Student’s t -test. Error bars represent s.e.m. Scale bars, 5 μM. Full size image To confirm that ALMS1-deficient cardiomyocytes proliferate with impaired cell cycle arrest, we differentiated cardiomyocytes from mouse embryonic stem cells (mESCs) that carry a cardiomyocyte-specific promoter ( Ncx1 ), which drives puromycin resistance, allowing efficient purification of cardiomyocytes (>98%) (ref. 24 ; Supplementary Fig. 3 ). By immunohistochemistry, we confirmed the presence of cardiomyocytes in pro-, meta-, ana- and telophase of mitosis after knockdown of Alms1 ( Fig. 5b–e ), demonstrating that these cardiomyocytes complete the cell cycle in vitro . In accordance with this observation, the amount PAK-positive cardiomyocytes was higher in ALMS1-deficient cardiomyocytes compared with control (0.41±0.09% versus 0.15±0.03%, mean±s.e.m., N =3, respectively, Student’s t -test, P <0.05; Fig. 5f ). To confirm that ALMS1 loss extends the proliferative window of cardiomyocytes, we treated puromycin-selected cardiomyocytes with Alms1 siRNA or control siRNA. After 48 h, we pulse-labeled cardiomyocytes with 5-ethynyl-2′-deoxyuridine (EdU) for 12 h. We observed an increase in EdU-positive cardiomyocytes after Alms1 knockdown compared with controls (13.6±1.0% versus 10.2±0.6%, mean±s.e.m., N =15, respectively, Student’s t -test, P <0.05) ( Fig. 5g ). During maturation, cardiomyocytes undergo karyokinesis (nuclear division) but not cytokinesis (cell division) and become terminally differentiated [25] . To exclude the possibility that the observed increase in EdU-positive uptake is due to karyokinesis and not cytokinesis, we counted cardiomyocytes 72 h after siRNA treatment and found that the number of cardiomyocytes was higher after Alms1 knockdown compared with control (51,915±1,821 cm −2 versus 46,696±1,311 cm −2 , mean±s.e.m., N =4, respectively, Student’s t -test, P <0.05) ( Fig. 5h ). Taken together, these results confirm that ALMS1 deficiency increases cardiomyocyte proliferation in vitro . Impaired cardiomyocyte cell cycle arrest in Alms1 Gt/Gt mice To investigate the role of ALMS1 in vivo , we used Alms1 Gt/Gt mice with truncated Alms1 mRNA and many characteristics of human Alström syndrome [26] . In mice, the maturation process from mono- to binucleate state occurs during postnatal days 5–10, resulting in 95–99% cardiomyocytes being binucleated and terminally differentiated at 10 days of age [21] , [25] . We therefore analysed mouse hearts at 15.5 days of age for persistent cardiomyocyte proliferation. To do this, we treated 15-day-old mice with a pulse dose of EdU, and 12 h later their hearts were isolated and EdU uptake in cardiomyocytes was analysed using the double-blinded quantification method described above. In the Alms1 Gt/Gt mutant mice, >8% of cardiomyocytes were EdU positive compared with very low levels in the wild-type littermate controls (8.3±0.91% versus 0.3±0.04%, mean±s.e.m., N =4, respectively, Student’s t -test, P <0.001; Fig. 6a–c ). Accordingly, we also observed a higher number of PH3-positive cardiomyocytes in homozygous Alms1 Gt/Gt mutant mice compared with their wild-type littermates (13.2±2.6 mm −2 compared with <1 mm −2 ; mean±s.e.m., N =3, Student’s t -test, P <0.01) ( Fig. 6d–f ). Additional staining demonstrated increased PAK-positive cardiomyocytes in the Alms1 Gt/Gt mice compared with wild-type controls (1.36±0.1 mm −2 versus 0.11±0.1 mm −2 , mean±s.e.m., N =3, Student’s t -test, respectively, P <0.001) ( Fig. 6g–i ). Importantly, we did not observe any difference in apoptosis (caspase-3-positive or terminal deoxynucleotidyl transferase dUTP nick end labeling-positive cells) between Alms1 Gt/Gt mutant mice and their littermate controls ( Supplementary Figs 4 and 5 ). 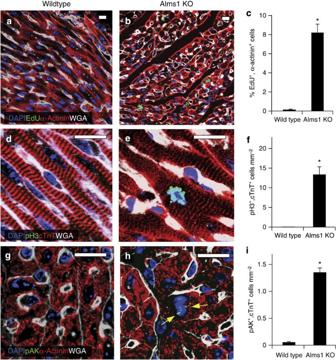Figure 6: Increased cardiomyocyte proliferation in homozygousAlms1Gt/Gtmutant mice. (a,b) Representative confocal images demonstrating EdU (green) incorporation inAlms1Gt/Gtversus wild-type littermate control mouse cardiac myocytes; α-sarcomeric actinin (red), WGA (white) and DAPI (blue). (c) Bar graph comparing cardiomyocyte EdU incorporation inAlms1Gt/Gtmutant (KO) versus wild-type littermate control mice (N=4 each). ‘*‘ refers toP<0.001 using unpaired Student'st-test. (d,e) Representative confocal images demonstrating PH3 (green) in a cardiomyocyte nucleus in aAlms1Gt/Gtmutant versus wild-type littermate control mouse, with cTnT (red), WGA (white) and DAPI (blue). (f) Comparison of the number of PH3-positive cardiomyocytes inAlms1Gt/Gt(KO) versus wild-type littermate control mice (N=3 each). ‘*‘ refers toP<0.01 using unpaired Student'st-test. (g,h) Representative confocal images demonstrating PAK staining (green) is present in a dividing cardiomyocyte nucleus in anAlms1Gt/Gtmouse (KO); DAPI (blue) highlights the nucleus, which is surrounded by α-sarcomeric actinin (red) to highlight cardiomyocytes and WGA (white) to identify cell boundaries. (i) Comparison of the number of PAK-positive cardiomyocytes inAlms1Gt/Gt(KO) versus wild-type controls. Scale bars, 10 μm. Error bars represent s.e.m.;N=3 each. ‘*‘ refers to P<0.001 using unpaired Student'st-test. Figure 6: Increased cardiomyocyte proliferation in homozygous Alms1 Gt/Gt mutant mice. ( a , b ) Representative confocal images demonstrating EdU (green) incorporation in Alms1 Gt/Gt versus wild-type littermate control mouse cardiac myocytes; α-sarcomeric actinin (red), WGA (white) and DAPI (blue). ( c ) Bar graph comparing cardiomyocyte EdU incorporation in Alms1 Gt/Gt mutant (KO) versus wild-type littermate control mice ( N =4 each). ‘*‘ refers to P <0.001 using unpaired Student's t -test. ( d , e ) Representative confocal images demonstrating PH3 (green) in a cardiomyocyte nucleus in a Alms1 Gt/Gt mutant versus wild-type littermate control mouse, with cTnT (red), WGA (white) and DAPI (blue). ( f ) Comparison of the number of PH3-positive cardiomyocytes in Alms1 Gt/Gt (KO) versus wild-type littermate control mice ( N =3 each). ‘*‘ refers to P <0.01 using unpaired Student's t -test. ( g , h ) Representative confocal images demonstrating PAK staining (green) is present in a dividing cardiomyocyte nucleus in an Alms1 Gt/Gt mouse (KO); DAPI (blue) highlights the nucleus, which is surrounded by α-sarcomeric actinin (red) to highlight cardiomyocytes and WGA (white) to identify cell boundaries. ( i ) Comparison of the number of PAK-positive cardiomyocytes in Alms1 Gt/Gt (KO) versus wild-type controls. Scale bars, 10 μm. Error bars represent s.e.m. ; N =3 each. ‘*‘ refers to P<0.001 using unpaired Student's t -test. Full size image Phenotypic characterization of Alms1 Gt/Gt at postnatal day 15.5 demonstrated that ALMS1-mutant mouse heart/body ratio was larger in Alms1 Gt/Gt mice ( N =7) compared to wild-type littermates ( N =16; 7.2±0.3 versus 6.4±0.2, mean±s.e.m., Student’s t -test, P <0.05; Fig. 7 ). In addition, Alms1 Gt/Gt cardiomyocytes were smaller compared with wild-type littermate controls (128.2±10.6 μM 2 versus 176.1±8.5 μM 2 , mean±s.e.m., N =4, Student’s t -test, P <0.01) ( Fig. 7 ), implying that cardiomyocyte number is increased in Alms1 Gt/Gt hearts. Together, these findings indicate that terminal differentiation is impaired in ALMS1-deficient cardiomyocytes, and that ALMS1-deficient cardiomyocytes remain proliferative beyond the normal window of postnatal cardiomyocyte cell cycle arrest. Alms1 levels in dividing cardiomyocytes obtained from proliferative mouse hearts (embryonic day 15.5) are relatively low, compared with levels at the beginning of the maturation process (postnatal day 6) when cytokinesis rapidly declines, suggesting that ALMS1 may be transcriptionally regulated during perinatal development ( Fig. 8 ). 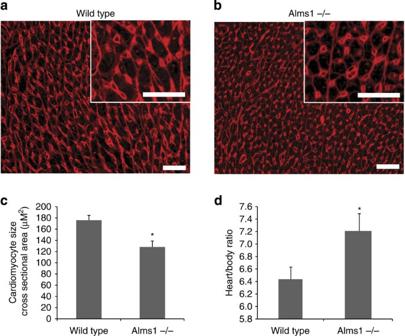Figure 7: Increased cardiomyocyte density and normalized heart size in homozygousAlms1Gt/Gtmutant mice. Representative images of (a) wild-type (WT) and (b)Alms1Gt/Gthearts stained with WGA (white) and cTnT (red); scale bars, 50 uM. (c) Measured cardiomyocyte cross sectional area,N=12 each; ‘*‘ indicatesP<0.01 using Student'st-test. (d) Heart/body weight ratios,N=16 for WT andN=7 forAlms1−/−; error bars represent s.e.m.; ‘*’ indicatesP<0.05 using Student’st-test. Figure 7: Increased cardiomyocyte density and normalized heart size in homozygous Alms1 Gt/Gt mutant mice. Representative images of ( a ) wild-type (WT) and ( b ) Alms1 Gt/Gt hearts stained with WGA (white) and cTnT (red); scale bars, 50 uM. ( c ) Measured cardiomyocyte cross sectional area, N =12 each; ‘*‘ indicates P <0.01 using Student's t -test. ( d ) Heart/body weight ratios, N =16 for WT and N =7 for Alms1 −/− ; error bars represent s.e.m. ; ‘*’ indicates P <0.05 using Student’s t -test. 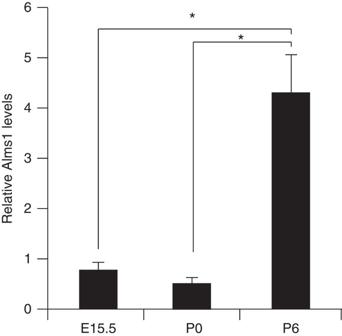Figure 8: Perinatal expression ofAlms1in murine cardiomyocytes. Murine GFP-positive cardiomyocytes were isolated from αMHC-GFP transgenic mice by fluorescence-activated cell sorting.Alms1mRNA levels were normalized toGapdh. RelativeAlms1mRNA levels at embryonic day 15.5 (E15.5;N=4) and postnatal day 0 (P0;N=4) were compared by student’st-test to postnatal days 5.5/6.5 (P5/6;N=10),P=0.02 andP=0.013, respectively. ‘*’ denotesP<0.05. There was no significant difference inAlms1expression between days E15.5 and P0; error bars indicate s.e.m. Full size image Figure 8: Perinatal expression of Alms1 in murine cardiomyocytes. Murine GFP-positive cardiomyocytes were isolated from αMHC-GFP transgenic mice by fluorescence-activated cell sorting. Alms1 mRNA levels were normalized to Gapdh . Relative Alms1 mRNA levels at embryonic day 15.5 (E15.5; N =4) and postnatal day 0 (P0; N =4) were compared by student’s t -test to postnatal days 5.5/6.5 (P5/6; N =10), P =0.02 and P =0.013, respectively. ‘*’ denotes P <0.05. There was no significant difference in Alms1 expression between days E15.5 and P0; error bars indicate s.e.m. Full size image We considered whether our findings could be due to an increased number of cardiac stem cells. However, we observed no difference in the number of c-kit+ or Sca-1+ cardiac stem cell markers in Alms1 Gt/Gt compared with littermates (both makers <1 cell per 225 μM 2 ). As cardiac stem cells differentiate, they may lose c-kit or Sca-1 markers. Thus, we cannot exclude that the increase in proliferating cardiomyocytes may arise in part from resident cardiac stem cells. Our data show that ALMS1 is a key molecule for cell cycle regulation in perinatal cardiomyocytes. ALMS1 is a component of the non-motile primary cilium, a subcellular organelle that projects from most cell types. Its presence is temporally associated with cellular quiescence with resorption during mitosis [27] . Induction of a longer cilium causes delay in G1/S transition, and ciliary disassembly increases S-phase [28] , [29] . Prior reports show that certain components of the primary cilium restrain canonical Wnt/β-catenin signalling that has an important role in cardiomyogenesis [30] , [31] . Deficiency of ALMS1 may activate Wnt/β-catenin signalling, thereby activating the transcription factor TCF/LEF (T-cell factor/lymphoid enhancer factor) and inducing transcription of genes that promote cell cycle proliferation [32] , [33] . Definitive proof of cardiomyocyte cytokinesis can be challenging. Proliferation markers, such as PH3, Ki67 and EdU, cannot discern karyokinesis from cytokinesis. Increased PAK staining in humans and mice with ALMS1 deficiency is consistent with increased cytokinesis, but it is insufficient. The increased density of cardiomyocytes in Alms1 -mutant mice and the increased number of cardiomyocytes with cell-counting studies after Alms1 knockdown are further supportive of amplified cardiomyocyte cytokinesis. However, the evidence for cytokinesis, and therefore the completion of mitosis, is inconclusive and warrants further investigation. Mitogenic cardiomyopathy is a very rare human phenotype, previously of unknown aetiology. Our finding of homozygous or compound heterozygous mutations in ALMS1 among all six affected infants from whom DNA was available suggests that this is the main cause. However, in each of these individuals, hearts were removed either at the time of transplantation due to end-stage heart failure or after death from heart failure [6] . Cardiomyopathy is found in approximately two-thirds of affected individuals, which suggests that other factors contribute to its development besides ALMS1 mutations [18] . When cardiomyopathy develops in infancy, it can precede other manifestations, at times obscuring the diagnosis of Alström syndrome, as among these six infants and as previously reported [19] . The cardiac function of the ALMS1-mutant mice is normal [26] . However, our findings do not rule out an injury response that contributes to myocyte proliferation in the context of an ALMS1 mutation. ALMS1 localizes to the centrosome that has a pivotal role in regulation of the cell cycle [34] , [35] . At postnatal day 15 (1 week beyond the normal window of postnatal cardiomyocyte cell cycle arrest), ALMS1-deficient mice display persistent cardiomyocyte proliferation, indicating that ALMS1-deficient cardiomyocytes may have an impaired ability to undergo cell cycle arrest. A similar finding was previously reported for the transcription factor MEIS1, although no direct link between MEIS1 and ALMS1 is currently known [5] . Throughout mitosis, ALMS1 localizes to the centrosomal spindle poles, and during late mitosis, ALMS1 localizes to the contractile ring and the cleavage furrow [36] . ALMS1 retains the centrosome cohesion protein C-NAP1, an important regulator of centrosome organization during mitosis. Depletion of ALMS1 reduces centrosomal levels of C-NAP1 and increases centrosome splitting, a key event for chromosomal division during anaphase [34] . In addition, ALMS1 interacts with several cytoskeleton-associated components that are necessary for the recycling of receptors to the plasma membrane, also referred to as endocytic trafficking [36] . During mitosis endocytic trafficking is repressed, as continued endocytosis may interfere with accurate chromosome segregation [37] , [38] , [39] . Interestingly, endocytic trafficking is significantly reduced in ALMS1-deficient cells [36] . Whether the impairment of terminal differentiation of cardiomyocyte proliferation is partly because of diminished endocytic trafficking remains unclear. Further investigation of this role of ALMS1 may identify novel and therapeutically important avenues to alter cardiomyocyte replication. Exome sequencing All human subjects (or their legal representative) signed informed consent, and the research was approved by the Johns Hopkins University Institutional Review Board. Genomic DNA was obtained from the proband’s dermal fibroblasts and from blood from each of the parents by the Gentra Puregene Tissue/Blood Kit (Qiagen). Genomic DNA (3 μg) was sheared using the Covaris S-2 instrument (Covaris) using the recommended settings according to the Agilent protocol (SureSelect Target enrichment System for Illumina Paired End and Multiplexed Sequencing Library v1.0) for a 150–200 bp fragment size. Libraries were prepared for targeted enrichment using the SPRIworks Fragment Library System I (200–400 bp size selection) according to Beckman-Coulter’s protocol (version 2.0). Adaptor ligated fragments were amplified according to the Agilent protocol for six cycles; 500 ng of amplified library was used in a whole-exome enrichment reaction with the SureSelect Human All Exon, 50 Mb product (Agilent WE). Samples were clustered one per flow cell lane using the Illumina cBot Paired End Cluster Generation Kit with v1 HiSeq flow cell (Illumina). Seventy-six base pairs paired-end sequencing was performed on the HiSeq2000 with TruSeq SBS v1 chemistry (Illumina). Intensity analysis and base calling were performed through the Illumina Real-Time Analysis software (version 1.7.48.0). Average sequence yield for the samples was 9.2 Gb having a quality value of Q30 or greater. Basecall files were converted from a binary format (BCL) to flat file format (qseq.txt) using the Illumina BCL Converter software (version 1.7.1). Basecall files were converted to fastq format, aligned with Burrows-Wheeler Aligner [40] version 0.5.7 to the GRCh37 human genome reference. Duplicate molecules were flagged with Picard version 1.26. Single nucleotide variants (SNVs) and indels were called using SAMtools [41] version 0.1.7. Only variant calls from the reference genome having a minimum depth of 10 × were considered for downstream analysis. In addition, for SNVs, only those calls where the root mean square of their read mapping qualities (RMS) >20 were considered, whereas for indels only those with an RMS >15 were considered. Samples were processed on the Illumina Infinium HumanOmniExpress (OE) beadchip to confirm family and gender relationships, and provide sample identity confirmation against the sequencing data. The mean on-bait coverage (regions covered by probes in the Agilent WE) was greater than 77 × for each sequencing experiment and >92% of on-bait bases had a depth >10 × . Overall concordance to genotypes for each sample was >99.5%. Greater than 93% of the OE heterozygote genotypes for each sample within the baited regions were called as variants against reference in the sequencing experiments. All remaining variants were annotated using the SeattleSeq Annotation Server build 6.03 (ref. 42 ). Variants present in dbSNP131 or the 1,000 genomes pilot April 2010 data set were filtered out. Only missense, nonsense or splice site compound heterozygotes present in the offspring, where one allele each was inherited from the parents, were considered. After this level of filtering, six compound missense heterozygotes and one compound heterozygote frameshift indel remained. Statistical analyses For all cellular and immunohistochemistry quantification, the unpaired two-tailed Student’s t -test, type II, was used for data analyses. P <0.05 was considered significant. Cell culture and analysis Mouse neonatal cardiomyocytes were isolated from newborn mouse hearts on PD0.5. Hearts were minced and digested with collagenase type II and pancreatase myocyte digestion buffer. To enrich for cardiomyocytes, dissociated cells were pre-plated by the conventional pre-plating method [22] , [43] . Enriched cardiomyocytes were cultured in Dulbecco’s Modified Eagle Medium (Gibco) supplemented with 20% horse serum and 2 mM GlutaMAX (Invitrogen) in 5% CO 2 . Cardiac fibroblasts were identified by their expression of the cardiac fibroblast marker Thy-1 (refs 22 , 23 ). mESCs carrying a puromycin resistance cassette driven by the cardiomyocyte-specific sodium-calcium exchanger 1 gene ( Ncx1 ) promoter [44] were maintained and cultured on gelatin-coated tissue culture dishes in standard maintenance medium (Glasgow minimum essential medium with 10% fetal bovine serum and 1,500 U leukemia inhibitory factor ml −1 (Millipore)), glutamax, sodium pyruvate and non-essential amino acids [45] . For differentiation, ESCs were allowed to form embryoid bodies in the IMDM/Ham-F12 (Cellgro) (3:1) supplemented with N2, B27, penicillin/streptomycin, 2 mM GlutaMAX, 0.05% BSA, 5 ng ml −1 L-ascorbic acid (Sigma‐Aldrich), α‐monothioglycerol (Sigma‐Aldrich). For mesoderm induction, embryoid bodies were dissociated and reaggregated in the presence of Activin A, bone morphogenetic protein-4 and vascular endothelial growth factor for 48 h (ref. 46 ). Cardiomyocytes were selected with Puromycin (2.5 μg ml −1 ) for 48 h (ref. 44 ), dissociated and counted using an automated cell counter (Scepter 2.0, Millipore). RNA suppression and cell cycle analysis Cardiomyocytes were transfected with Lipofectamine RNAiMAX (Invitrogen). For Alms1 knockdown experiments, Alms1 ON-TARGETplus SMARTpool and Alms1 siRNA (Ambion) or scrambled siRNA oligonucleotides (Dharmacon) and siRNA negative control (Ambion) were used at a final concentration of 100 nM for cell transfection. Forty-eight hours after transfection, cells were fixed and stained for flow cytometry with the following antibodies: anti-Ki67 (1:200, cat. no. ab15580, Abcam), -PAK A/B/C (1:200, cat. no. 2914S, Cell Signaling), -PH3 (1:400, cat. no. ab5176, Abcam), -cTnT (1:500, cat. no. 13-11, Thermo Scientific), -Thy1-APC (1:200, cat. no. 17-0902-81, eBiosciences), with secondary detection using the appropriate Alexa Fluor-conjugated antibody (1:400, Invitrogen). For S-phase analysis, cardiomyocytes were treated with 100 μM EdU for 30 min before fixation and stained using Click-iT EdU cell proliferation kit (Invitrogen). For cell cycle analysis, dissociated cardiomyocytes were incubated for 30 min with 5 μM Vybrant Dye Cycle Ruby Stain (Invitrogen). For EdU analysis, cells were treated with 100 μM EdU for 30 min before isolation and fixation. EdU incorporation was detected using Click-it EdU Alexa Fluor Imaging Kit (Invitrogen) according to manufacturer’s protocol. Cells were analysed on an Accuri C6 flow cytometer (BD Biosciences) using FlowJo software (Treestar). Mice The Alms1 Gt/Gt mice (B6.129P2- Alms1 Gt(XH152)Byg /Pjn) used in this study were generated from gene-trapped ESCs (MMRC no. 008633) (refs 26 , 47 ). Mice were fed ad libitum a 4K54 diet (PMI Nutrition International, St Louis, MO, USA) and provided an unlimited access to water in a temperature/humidity controlled setting with a 12-h light/dark cycle at The Jackson Laboratory Research Animal Facility. All mouse protocols used in this study were approved by the JAX institutional Animal Care and Use Committee. Mouse hearts were extracted from mice killed by CO 2 asphyxiation and allowed to contract in phosphate-buffered saline for 5–10 min and immediately placed in 4% paraformaldehyde at 4 °C overnight. Subsequently, tissues were embedded in paraffin, sectioned and immunostained as previously reported [48] . The αMHC promoter-driven EGFP-IRES-puromycin transgenic mice (αMHC-GFP), in which only cardiomyocytes express the GFP facilitate rapid and efficient isolation of cardiomyocytes [23] . Hearts from these mice were dissociated using collagense II/TrypLE. GFP+ cardiomyocytes were isolated by fluorescence-activated cell sorting using an SH800 sorter (Sony Biotechnology). Histology and immunohistochemistry Paraffin-embedded heart sections were rehydrated, followed by antigen retrieval. Immunostaining was performed on cultured cardiomyocytes and mouse cardiac tissue with primary antibodies against Ki67, cTnT, α-sarcomeric actinin, PH3, PAK A/B/C or activated caspase-3 followed by secondary detection with appropriate Alexa Fluor-conjugated antibodies. Additional staining was done with WGA conjugated with Alexa Fluor-647 dye to show cell boundaries. Analyses using confocal microscopy were quantified in a blinded fashion by two independent observers. All images were acquired with a Zeiss LSM 510 Meta Confocal system and analysed with Volocity imaging software. Puromycin-selected cardiomyocytes were fixed in 4% formaldehyde. Cardiomyocytes were permeabilized with 0.5% saponin/phosphate-buffered saline and stained with antibodies against cTnT or isotype control antibodies followed the appropriate Alexa Fluor-conjugated antibody (Invitrogen). Determination of cardiomyocyte density and size Postnatal day 15 wild-type and Alms1 Gt/Gt mouse hearts were fixed with methanol, paraffin embedded, sectioned, deparaffinized, rehydrated and subjected to citrate-based heat-mediated antigen retrieval. Slides were incubated with 5 μg ml −1 Alexa Fluor-647-conjugated WGA (Invitrogen) overnight at 4 °C and mounted in Vectashield containing 4′,6-diamidino-2-phenylindole (DAPI) (Vector Labs, CA, USA). Image acquisition was performed on an EVOS epifluorescence microscope (Life Technologies). Cardiomyocyte cross sectional area was measured using an automated algorithm with National Institutes of Health (NIH) Image J 1.47i software analysing 300–600 cells from 3–4 areas per mouse heart. Quantitative quantitative reverse transcriptase–PCR RNA was extracted with TRIzol (Invitrogen). Reverse transcriptase–quantitative PCR was performed using the Superscript III first-strand synthesis system (Invitrogen) followed by use of TaqMan probes on the ABI 7900HT (Applied Biosystems) according to the manufacturer's protocols. Optimized primers from TaqMan Gene Expression Array were used. Expression levels were normalized to Gapdh expression. All samples were run at least in triplicate. Real-time PCR data were normalized and standardized with SDS2.2 software. Quantitative fluorescence To measure nuclear DNA content, 20-μm-thick histology sections of the proband’s heart were stained with DAPI. Using a Zeiss LSM 510 Meta confocal microscope and Zen software for image acquisition, the nuclear DNA content of cardiac myocytes was assayed by measuring the total fluorescence from each selected nucleus with Volocity imaging software. Background fluorescence was excluded before image acquisition using Zen software. Nuclei in contact with the edges of the image stack or touching other nuclei were excluded. The total DAPI fluorescence signal associated with diploid status was designated 1 in non-proliferating cells (negative for PH3 staining). The DNA content of proliferating cardiomyocytes (positive for PH3 staining) was compared with non-proliferating cells and displayed as a ratio of the total quantitative fluorescence. A value of 2 would indicate cells that have a full duplication of nuclear DNA before karyokinesis. Accession codes: Whole-exome sequence data for the proband has been deposited in the GenBank dbGaP (database of Genotypes and Phenotypes) database under the accession code phs000711.v1.p1. Sequence data for ALMS1 from additional patients have been deposited in the GenBank nucleotide core database under the accession codes AB905563 to AB905565 . How to cite this article: Shenje, L. T. et al. Mutations in Alström protein impair terminal differentiation of cardiomyocytes. Nat. Commun. 5:3416 doi: 10.1038/ncomms4416 (2014).